A metabolic stress-inducible miR-34a-HNF4α pathway regulates lipid and lipoprotein metabolism Non-alcoholic fatty liver disease (NAFLD) is one of the most common liver diseases, but its underlying mechanism is poorly understood. Here we show that hepatocyte nuclear factor 4α (HNF4α), a liver-enriched nuclear hormone receptor, is markedly inhibited, whereas miR-34a is highly induced in patients with non-alcoholic steatohepatitis, diabetic mice and mice fed a high-fat diet. miR-34a is essential for HNF4α expression and regulates triglyceride accumulation in human and murine hepatocytes. miR-34a inhibits very low-density lipoprotein secretion and promotes liver steatosis and hypolipidemia in an HNF4α-dependent manner. As a result, increased miR-34a or reduced HNF4α expression in the liver attenuates the development of atherosclerosis in Apoe −/− or Ldlr −/− mice. These data indicate that the miR-34a-HNF4α pathway is activated under common conditions of metabolic stress and may have a role in the pathogenesis of NAFLD and in regulating plasma lipoprotein metabolism. Targeting this pathway may represent a novel approach for the treatment of NAFLD. Obesity, diabetes and insulin resistance are common risk factors for non-alcoholic fatty liver disease (NAFLD) [1] , [2] , [3] , one of the most common liver diseases worldwide. In the United States, up to 25% of the population have NAFLD [4] , [5] . NAFLD initiates from simple steatosis, which may progress to non-alcoholic steatohepatitis (NASH) after multiple ‘hits’, including inflammatory mediators, reactive oxygen species (ROS), and so on [4] , [6] , [7] . NASH may further progress to liver cirrhosis and hepatocellular carcinoma. So far, the mechanism underlying the pathogenesis of NAFLD is poorly understood. Therefore, current treatment of NAFLD is limited to management of associated syndrome, such as diabetes and obesity [8] , [9] . Hepatocyte nuclear factor 4α (HNF4α) is a nuclear hormone receptor that plays an important role in both development and adult physiology. It is highly expressed in the liver, with lower levels in the kidney, intestine and pancreatic β cells [10] , [11] . HNF4α has a highly conserved DNA binding domain and a ligand-binding domain. Structural analysis of HNF4α indicates that C14–C18 long-chain fatty acids are tightly bound to the hydrophobic pocket of HNF4α and could not be dissociated from the receptor under non-denaturing conditions [12] , [13] . As such, HNF4α is constitutively active. HNF4α controls the basal expression of many genes involved in bile acid, lipid, glucose and drug metabolism. Loss-of-function mutations in human HNF4α cause maturity-onset diabetes of the young type 1 (MODY1), characterized by autosomal dominant inheritance, early-onset diabetes and pancreatic β-cell dysfunction [14] . The diabetes phenotype appears to result from reduced glucose-stimulated insulin secretion in the pancreas [15] . In addition to the diabetes phenotype, patients with MODY1 also have decreased plasma triglyceride (TG) and cholesterol levels [16] , [17] , [18] , likely as a result of impaired very low-density lipoprotein (VLDL) secretion in the liver [19] . Consistent with the reduced VLDL secretion, we and others have shown that loss of hepatic HNF4α results in fatty liver and hypolipidemia in mice [19] , [20] . MicroRNAs (miRNAs) are small non-coding RNA molecules that regulate gene expression post-transcriptionally via binding to the 3′-untranslated region (3′UTR) of mRNA. miRNAs have emerged as important regulators of cell proliferation, inflammation and metabolism. Recent studies have shown that hepatic miRNAs may have an important impact on lipid and lipoprotein metabolism [21] , [22] , [23] . In this report, we investigate the role of the miR-34a-HNF4α pathway in the pathogenesis of human NAFLD and in plasma lipid and lipoprotein metabolism. Our data show that this pathway is activated in both NASH patients and diabetic or high-fat diet (HFD)-fed mice. We then investigate whether and how this pathway regulates hepatic and plasma lipid and/or lipoprotein metabolism. Finally, we explore which metabolic cues trigger the activation of this pathway. Our data suggest that the miR-34a-HNF4α pathway may be an attractive target for treatment of human NAFLD. Inverse regulation of HNF4α and miR-34a expression in vivo We and others have previously shown that loss of hepatic HNF4α causes fatty liver in mice [19] , [20] . As HNF4α is highly conserved between humans and rodents, we explored the role of HNF4α in the development of human NAFLD. As compared with the normal subjects, NASH patients had increased levels of hepatic TG ( Fig. 1a ) and cholesterol ( Fig. 1b ). Remarkably, hepatic HNF4α mRNA levels were reduced by 80% ( Fig. 1c ) and HNF4α protein levels were almost undetectable ( Fig. 1d and Supplementary Fig. 1a ) in NASH patients. 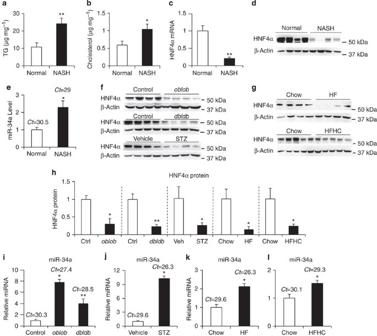Figure 1: Hepatic HNF4α and miR-34a expression is inversely regulated in NASH patients and diabetic or HFD-fed mice. (a–e) Hepatic levels of TG (a) cholesterol (b)Hnf4αmRNA (c) HNF4α protein (d) andmiR-34a(e) were determined in normal individuals or NASH patients (n=8). (f–h) Hepatic HNF4α protein levels were determined using western blots in diabeticob/obordb/dbmice (f;n=5) or STZ-treated mice (f;n=6), high-fat diet (HFD)-fed mice (g;n=5) or high-fat, high-cholesterol (HFHC) diet-fed mice (g;n=8). Protein levels were quantified by ImageJ (h). (i–l) HepaticmiR-34alevels were quantified inob/obordb/dbmice (i) STZ-treated mice (j) HFD-fed mice (k) or HFHC diet-fed mice (l). Results are shown as mean±s.e.m. Two-sided Student’st-test was performed. *P<0.05. **P<0.01. Consistent with a marked reduction in hepatic HNF4α expression, a number of HNF4α target genes were also significantly reduced in NASH patients ( Supplementary Table 1 ). miRNAs have been shown to play a role in the development of NAFLD [24] , [25] . In the livers of NASH patients, miR-34a ( Fig. 1e ), but not miR-19b or miR-27b ( Supplementary Fig. 1b ), was induced by >2-fold. Figure 1: Hepatic HNF4α and miR-34a expression is inversely regulated in NASH patients and diabetic or HFD-fed mice. ( a–e ) Hepatic levels of TG ( a ) cholesterol ( b ) Hnf4α mRNA ( c ) HNF4α protein ( d ) and miR-34a ( e ) were determined in normal individuals or NASH patients ( n =8). ( f–h ) Hepatic HNF4α protein levels were determined using western blots in diabetic ob / ob or db / db mice ( f ; n =5) or STZ-treated mice ( f ; n =6), high-fat diet (HFD)-fed mice ( g ; n =5) or high-fat, high-cholesterol (HFHC) diet-fed mice ( g ; n =8). Protein levels were quantified by ImageJ ( h ). ( i–l ) Hepatic miR-34a levels were quantified in ob / ob or db / db mice ( i ) STZ-treated mice ( j ) HFD-fed mice ( k ) or HFHC diet-fed mice ( l ). Results are shown as mean±s.e.m. Two-sided Student’s t -test was performed. * P <0.05. ** P <0.01. Full size image NAFLD is often associated with obesity, diabetes and insulin resistance. Therefore, we investigated hepatic expression of HNF4α and miR-34a in diabetes and HFD-induced obesity. In ob / ob or db / db mice (type 2 diabetes models), streptozotocin (STZ)-treated mice (a type 1 diabetes model), HFD-fed mice or high-fat/high-cholesterol (HFHC) diet-fed mice, hepatic HNF4α protein levels were decreased by 75–85% ( Fig. 1f–h and Supplementary Fig. 1c ), whereas hepatic miR-34a levels were induced by up to 10-fold ( Fig. 1i–l ). In these mice, hepatic mRNA levels of Hnf4α ( Supplementary Fig. 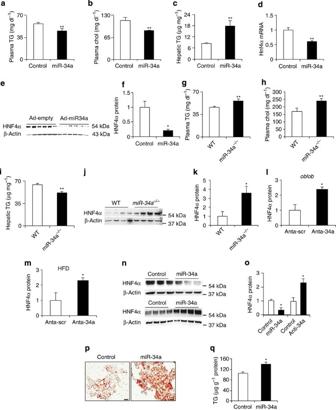Figure 2: miR-34a regulates lipid metabolism and inhibits HNF4α expression in mice and HepG2 cells. (a–f) C57BL/6 mice were injected i.v. with either Ad-empty (control) or Ad-miR-34a (miR-34a) (n=6). After 7 days, plasma TG (a) cholesterol (chol;b) and hepatic TG (c) levels were determined. HepaticHnf4αmRNA level was quantified by qRT-PCR (d). Hepatic protein levels were determined by western blots (e) and then quantified (f). (g–k) Wild-type andmiR-34a−/−mice were fed a Western diet for 12 weeks (n=5). Plasma TG (g) plasma cholesterol (h) and hepatic TG levels (I) were determined. Hepatic protein levels were determined by western blotting (j) and HNF4α protein levels quantified (k). (l,m)ob/obmice (l) or HFD-fed mice (m) were injected i.v. with anta-scr (scramble antagomir) or anta-miR-34a (miR-34a antagomir) once every 6 days (10 mg kg−1) (n=4–5). After three injections, hepatic HNF4α protein levels were determined. (n,o) HepG2 cells were treated with Ad-empty (control), Ad-miR-34a or Ad-anti-miR-34a (anti-miR-34a). After 48 h, protein levels were determined by western blotting (n) and then quantified (o) (n=3). (p,q) HepG2 cells were infected with Ad-empty or Ad-miR-34a for 48 h. Neutral lipids were stained by oil red O (p) and TG levels quantified (q) (n=6). The transfection assays were repeated once and similar results were obtained. Scale bar, 20 μm. Values are expressed as mean±s.e.m. Two-sided Student’st-test was performed. *P<0.05, **P<0.01. 1d ) or some Hnf4α target genes ( Supplementary Table 2 ) were reduced or unchanged and hepatic miR-19b or miR-27b expression did not alter ( Supplementary Fig. 1e ). Finally, the data from Northern blot assays confirmed that hepatic miR-34a was overexpressed in these models ( Supplementary Fig. 2a–c ). Together, these data indicate that hepatic HNF4α and miR-34a are inversely regulated in response to common metabolic stress. miR-34a regulates HNF4α expression and lipid metabolism To determine whether miR-34a regulates HNF4α expression and/or lipid metabolism, we injected adenoviruses expressing miR-34a (Ad-miR-34a) or Ad-empty (control) to C57BL/6 mice. Overexpression of miR-34a reduced plasma TG ( Fig. 2a ) and cholesterol ( Fig. 2b ) levels, increased hepatic TG levels by >2-fold ( Fig. 2c ) but had no effect on hepatic cholesterol levels ( Supplementary Fig. 3 ). Overexpression of miR-34a also significantly reduced hepatic Hnf4α mRNA levels by 40% ( Fig. 2d ) and HNF4α protein levels by >75% ( Fig. 2e,f ). Consistent with the gain-of-function data, miR-34a −/− mice had increased plasma levels of TG ( Fig. 2g ) and cholesterol ( Fig. 2h ), decreased hepatic TG levels ( Fig. 2i ) and a 3.6-fold increase in hepatic HNF4α protein levels ( Fig. 2j,k ). A >3-fold increase in hepatic HNF4α protein levels was also observed in chow- or HFD-fed miR-34a −/− mice ( Supplementary Fig. 4a–d ). When ob / ob mice or HFD-fed mice were treated with an miR-34a antagomir, hepatic miR-34a levels were reduced by 84% and HNF4α protein levels were increased by >2-fold ( Fig. 2l,m and Supplementary Fig. 5a–d ). These gain- and loss-of-function data demonstrate that miR-34a regulates lipid metabolism and hepatic HNF4α expression in mice. Figure 2: miR-34a regulates lipid metabolism and inhibits HNF4α expression in mice and HepG2 cells. ( a–f ) C57BL/6 mice were injected i.v. with either Ad-empty (control) or Ad-miR-34a (miR-34a) ( n =6). After 7 days, plasma TG ( a ) cholesterol (chol; b ) and hepatic TG ( c ) levels were determined. Hepatic Hnf4α mRNA level was quantified by qRT-PCR ( d ). Hepatic protein levels were determined by western blots ( e ) and then quantified ( f ). ( g – k ) Wild-type and miR-34a −/− mice were fed a Western diet for 12 weeks ( n =5). Plasma TG ( g ) plasma cholesterol ( h ) and hepatic TG levels ( I ) were determined. Hepatic protein levels were determined by western blotting ( j ) and HNF4α protein levels quantified ( k ). ( l , m ) ob / ob mice ( l ) or HFD-fed mice ( m ) were injected i.v. with anta-scr (scramble antagomir) or anta-miR-34a (miR-34a antagomir) once every 6 days (10 mg kg −1 ) ( n =4–5). After three injections, hepatic HNF4α protein levels were determined. ( n , o ) HepG2 cells were treated with Ad-empty (control), Ad-miR-34a or Ad-anti-miR-34a (anti-miR-34a). After 48 h, protein levels were determined by western blotting ( n ) and then quantified ( o ) ( n =3). ( p , q ) HepG2 cells were infected with Ad-empty or Ad-miR-34a for 48 h. Neutral lipids were stained by oil red O ( p ) and TG levels quantified ( q ) ( n =6). The transfection assays were repeated once and similar results were obtained. Scale bar, 20 μm. Values are expressed as mean±s.e.m. Two-sided Student’s t -test was performed. * P <0.05, ** P <0.01. Full size image In HepG2 cells, a human hepatoma cell line, overexpression of miR-34a reduced HNF4α protein levels by 66%, whereas inhibition of miR-34a expression by anti-miR-34a increased HNF4α expression by 2.2-fold ( Fig. 2n,o ). Consistent with a role of miR-34a in regulating lipid metabolism in mice, overexpression of miR-34a increased TG accumulation in HepG2 cells ( Fig. 2p,q ). Thus, the data of Fig. 2 demonstrate that miR-34a regulates HNF4α expression and lipid metabolism in both human and mouse hepatocytes. miR-34a regulates lipid metabolism by inhibition of HNF4α To determine how miR-34a regulates lipid metabolism, we analysed hepatic gene expression. miR-34a inhibited a number of genes involved in lipid metabolism, including Hnf4α , microsomal triglyceride transfer protein ( Mtp ), ApoB , sterol regulatory element-binding protein 1c ( Srebp-1c ), acetyl-CoA carboxylase 1 ( Acc1 ), Acc2 and HMG-CoA reductase ( Hmgcr ) ( Fig. 3a ). miR-34a also reduced MTP and ApoB protein levels ( Fig. 3b,c and Supplementary Fig. 6a ) and MTP activity ( Supplementary Fig. 6b ). In contrast, loss of miR-34a increased MTP activity ( Supplementary Fig. 6c ). Consistent with the latter data, miR-34a inhibited VLDL secretion ( Fig. 3d ). Interestingly, overexpression or loss of miR-34a had no effect on de novo lipogenesis ( Supplementary Fig. 7 ). 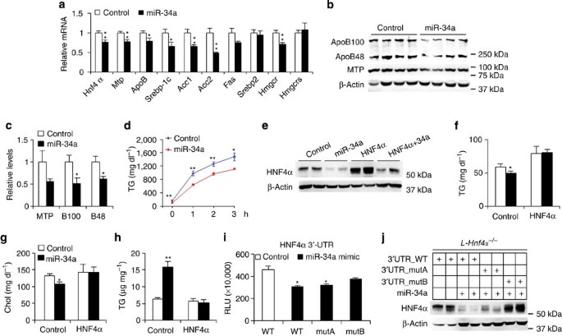Figure 3: miR-34a regulation of VLDL secretion and lipid metabolism depends on inhibition of hepatic HNF4α. (a–c) C57BL/6 mice were i.v. injected with Ad-empty or Ad-miR-34a (n=6). Hepatic mRNA (a) and protein levels (b,c) were quantified. B100, ApoB100. B48, ApoB48. (d) VLDL secretion was determined in C57BL/6 mice after i.p. injection of Tyloxapol (50 mg kg−1) (n=6). (e–h) C57BL/6 mice were injected i.v. with Ad-empty, Ad-miR-34a, Ad-HNF4α or Ad-miR-34a+Ad-HNF4α (n=7). Hepatic protein levels (e) plasma TG (f) plasma cholesterol (g) and hepatic TG levels (h) were determined. (i) HepG2 cells were transfected with a control mimic or miR-34a mimic, together with a pMIR-Report construct containing wild-type or mutant 3′ UTR of HNF4α (n=4). After 36 h, luciferase activity was determined and normalized to β-gal activity. MutA and mutB stand for the first or second mutant binding site for miR-34a, respectively. (j) Liver-specificHnf4α−/−mice were injected i.v. with Ad-HNF4α-3′UTR (3′UTR_WT), Ad-HNF4α-3′UTR_mutA (3′UTR_mutA) or Ad-HNF4α-3′UTR_mutB (3′UTR_mutB) plus or minus Ad-miR-34a. After 7 days, hepatic protein levels were determined. WT=wild type. Values are expressed as mean±s.e.m. Two-sided Student’st-test was performed. *P<0.05, **P<0.01. Figure 3: miR-34a regulation of VLDL secretion and lipid metabolism depends on inhibition of hepatic HNF4α. ( a – c ) C57BL/6 mice were i.v. injected with Ad-empty or Ad-miR-34a ( n =6). Hepatic mRNA ( a ) and protein levels ( b , c ) were quantified. B100, ApoB100. B48, ApoB48. ( d ) VLDL secretion was determined in C57BL/6 mice after i.p. injection of Tyloxapol (50 mg kg −1 ) ( n =6). ( e – h ) C57BL/6 mice were injected i.v. with Ad-empty, Ad-miR-34a, Ad-HNF4α or Ad-miR-34a+Ad-HNF4α ( n =7). Hepatic protein levels ( e ) plasma TG ( f ) plasma cholesterol ( g ) and hepatic TG levels ( h ) were determined. ( i ) HepG2 cells were transfected with a control mimic or miR-34a mimic, together with a pMIR-Report construct containing wild-type or mutant 3′ UTR of HNF4α ( n =4). After 36 h, luciferase activity was determined and normalized to β-gal activity. MutA and mutB stand for the first or second mutant binding site for miR-34a, respectively. ( j ) Liver-specific Hnf4α −/− mice were injected i.v. with Ad-HNF4α-3′UTR (3′UTR_WT), Ad-HNF4α-3′UTR_mutA (3′UTR_mutA) or Ad-HNF4α-3′UTR_mutB (3′UTR_mutB) plus or minus Ad-miR-34a. After 7 days, hepatic protein levels were determined. WT=wild type. Values are expressed as mean±s.e.m. Two-sided Student’s t -test was performed. * P <0.05, ** P <0.01. Full size image A deficiency in hepatic HNF4α causes fatty liver and hypolipidemia by reducing VLDL secretion [20] , [21] . The data of Figs 2 and 3a–d suggest that miR-34a regulates lipid metabolism likely through inhibition of HNF4α. To test this hypothesis, we overexpressed Hnf4α in mice infected with Ad-miR-34a to normalize hepatic HNF4α protein expression to the levels seen in the control mice ( Fig. 3e ). Hepatic overexpression of miR-34a reduced plasma levels of TG ( Fig. 3f ) and cholesterol ( Fig. 3g ) and increased hepatic TG levels ( Fig. 3h ) in the control mice. However, these changes were abolished when hepatic HNF4α protein expression was normalized ( Fig. 3f-h ). These data demonstrate that miR-34a regulates hepatic and plasma lipid metabolism through inhibition of hepatic HNF4α. To understand how miR-34a regulates HNF4α expression, we investigated whether miR-34a binds to the 3′UTR of HNF4α . There are two highly conserved miR-34a binding sites in both human and murine 3′UTRs of HNF4α ( Supplementary Fig. 8a,b ). As shown in Fig. 3i , an miR-34a mimic significantly repressed the activity of a luciferase promoter linked to the Hnf4α 3′UTR, and this repression was abolished when the second binding site for miR-34a (mutB) was mutated. To confirm the in vitro data, we overexpressed Hnf4α coding region plus wild type or mutant 3′UTR in liver-specific Hnf4α −/− mice. Overexpression of miR-34a markedly reduced exogenous HNF4α protein levels when the Hnf4α coding region was linked to the wild-type 3′UTR or 3′UTR with mutations in first binding site for miR-34a (mutA), and this reduction was abolished when the Hnf4α coding region was linked to 3′UTR with mutB ( Fig. 3j ). Thus, our in vitro and in vivo data demonstrate that miR-34a inhibits Hnf4α expression through binding to the second binding site of the 3′UTR. Hepatic HNF4α regulates atherogenesis and energy metabolism Loss-of-function mutations in HNF4α cause hypolipidemia in MODY patients. So far, it is unknown whether MODY1 patients are protective against the development of atherosclerosis. Given that hepatic HNF4α is markedly downregulated under various metabolic stress ( Fig. 1 ), we investigated the effect of acute versus chronic loss of hepatic HNF4α on the development of atherosclerosis. Acute knockdown of hepatic Hnf4α by shRNA in Apoe −/− mice for 3 weeks caused a >50% reduction in plasma total cholesterol levels and an ∼ 30% reduction in plasma TG on a Western diet ( Supplementary Fig. 9a–c ). Analysis of plasma lipoprotein profiles by fast protein liquid chromatography (FPLC) indicated that loss of hepatic Hnf4α reduced plasma VLDL cholesterol and LDL cholesterol ( Fig. 4a ) and VLDL TG ( Fig. 4b ). Consistent with the changes in plasma lipids and lipoproteins, acute knockdown of hepatic Hnf4α in Apoe −/− mice reduced aortic lesion sizes by >50% ( Fig. 4c and Supplementary Fig. 9d ). In addition, loss of hepatic Hnf4α in Apoe −/− mice increased hepatic TG accumulation ( Fig. 4d ) and reduced MTP and ApoB protein expression ( Supplementary Fig. 9e ). These data indicate that acute loss of hepatic HNF4α reduces the development of atherosclerosis in Apoe −/− mice. 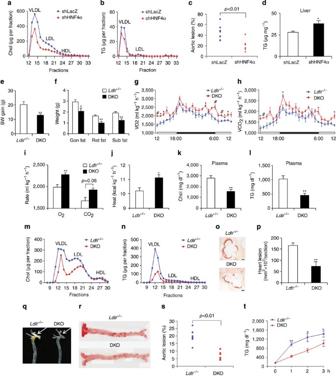Figure 4: Loss of hepatic HNF4α improves energy homeostasis and protects against atherosclerosis. (a–d)Apoe−/−mice were fed a Western diet for 4 weeks, followed by injection of Ad-shLacZ or Ad-shHNF4α (n=6). Three weeks following adenoviral injection, plasma cholesterol (a) and TG (b) lipoprotein profiles were determined.En faceaortic lesion sizes were analysed (c) and hepatic TG levels quantified (d). (e–t)Hnf4αfl/flLdlr−/−(Ldlr−/−) mice andHnf4αfl/flAlb-CreLdlr−/−(DKO) mice were fed a Western diet for 16 weeks (n=6). Body weight gain (e) and body fat content from gonadal (gon) fat, retroperitoneal (ret) fat and subcutaneous (sub) fat (f) were determined. O2consumption (g,i) CO2production (h,i) and heat production (j) were assessed by CLAMS. Plasma cholesterol (k) TG (l) cholesterol lipoprotein profile (m) and TG lipoprotein profile (n) were analysed. Aortic root was stained by oil red O (o) and lesion size quantified (p). Aorta was isolated (q) stained by oil red O (r) and theen facelesion size quantified (s). VLDL secretion was performed when mice were fed a Western diet for 12 weeks (t). In (q) the arrow shows the location of the brachiocephalic artery. Scale bar, 200 μm. Values are expressed as mean±s.e.m. Two-sided Student’st-test was performed. *P<0.05, **P<0.01. Figure 4: Loss of hepatic HNF4α improves energy homeostasis and protects against atherosclerosis. ( a – d ) Apoe −/− mice were fed a Western diet for 4 weeks, followed by injection of Ad-shLacZ or Ad-shHNF4α ( n =6). Three weeks following adenoviral injection, plasma cholesterol ( a ) and TG ( b ) lipoprotein profiles were determined. En face aortic lesion sizes were analysed ( c ) and hepatic TG levels quantified ( d ). ( e–t ) Hnf4α fl/fl Ldlr −/− ( Ldlr −/− ) mice and Hnf4α fl/fl Alb-CreLdlr −/− (DKO) mice were fed a Western diet for 16 weeks ( n =6). Body weight gain ( e ) and body fat content from gonadal (gon) fat, retroperitoneal (ret) fat and subcutaneous (sub) fat ( f ) were determined. O 2 consumption ( g , i ) CO 2 production ( h , i ) and heat production ( j ) were assessed by CLAMS. Plasma cholesterol ( k ) TG ( l ) cholesterol lipoprotein profile ( m ) and TG lipoprotein profile ( n ) were analysed. Aortic root was stained by oil red O ( o ) and lesion size quantified ( p ). Aorta was isolated ( q ) stained by oil red O ( r ) and the en face lesion size quantified ( s ). VLDL secretion was performed when mice were fed a Western diet for 12 weeks ( t ). In ( q ) the arrow shows the location of the brachiocephalic artery. Scale bar, 200 μm. Values are expressed as mean±s.e.m. Two-sided Student’s t -test was performed. * P <0.05, ** P <0.01. Full size image To determine whether chronic loss of hepatic HNF4α has a similar effect on atherosclerosis, we crossed HNF4α fl/fl mice with Ldlr −/− mice. These mice were then crossed with albumin-Cre mice to generate double-knockout (DKO) mice deficient in both Ldlr and hepatic Hnf4α as well as control ( Ldlr −/− HNF4α fl/fl ) mice. As compared with the control mice, the DKO mice had increased food intake ( Supplementary Fig. 10a ) but gained less body weight ( Fig. 4e ) and body fat content ( Fig. 4f ), and had increased O 2 consumption and CO 2 production ( Fig. 4g–i ) as well as heat production ( Fig. 4j ). Mechanistically, DKO mice had increased Cpt1b expression in the liver ( Supplementary Fig. 10b,c ), suggesting that hepatic fatty acid oxidation may be increased in these mice. In addition, the DKO mice had a >50% reduction in plasma cholesterol ( Fig. 4k ) and TG ( Fig. 4l ), and these changes were due to a marked reduction in plasma VLDL cholesterol and LDL cholesterol ( Fig. 4m ) and VLDL TG ( Fig. 4n ), respectively. ln agreement with the change in plasma lipid profile, DKO mice had a >50% reduction in the lesion size of aortic root ( Fig. 4o,p ), brachiocephalic artery ( Fig. 4q ) or aorta ( Fig. 4r,s ). Finally, consistent with a role of hepatic HNF4α in controlling VLDL secretion, DKO mice had reduced VLDL secretion ( Fig. 4t ). Thus, chronic loss of hepatic Hnf4α in Ldlr −/− mice increases energy expenditure and protects against the development of atherosclerosis. Hepatic miR-34a inhibits atherogenesis in Ldlr −/− mice The finding that miR-34a regulates lipid metabolism through inhibition of HNF4α ( Fig. 3 ) led us to ask whether miR-34a also regulates the development of atherosclerosis. Overexpression of miR-34a in Western diet-fed Ldlr −/− mice reduced plasma total cholesterol ( Fig. 5a ) and TG levels ( Fig. 5b ). The data from FPLC analysis showed that miR-34a reduced the levels of VLDL and LDL cholesterol ( Fig. 5c ) as well as VLDL TG ( Fig. 5d ). As a result, overexpression of miR-34a in the liver reduced the atherosclerotic lesion size by >50% in both the aortic root ( Figs 5e,f ) and aorta ( Fig. 5g,h ) of Ldlr −/− mice. In the liver, overexpression of miR-34a in Ldlr −/− mice inhibited hepatic HNF4α, ApoB100 and ApoB48 expression ( Fig. 5i ) and increased hepatic TG levels ( Supplementary Fig. 11 ). Thus, either overexpression of hepatic miR-34a ( Fig. 5 ) or inhibition of hepatic HNF4α ( Fig. 4 ) can provide protection against the development of atherosclerosis. 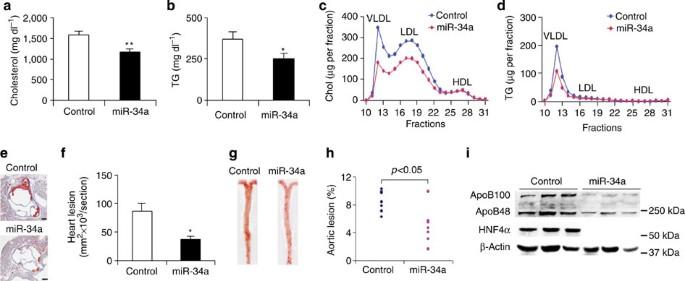Figure 5: miR-34a reduces the development of atherosclerosis inLdlr−/−mice. Ldlr−/−mice were fed a Western diet for a total of 7 weeks (n=6). At the end of week 4, the mice were injected i.v. with Ad-empty or Ad-miR-34a. Plasma cholesterol (a) TG (b) cholesterol lipoprotein profile (c) and TG lipoprotein profile (d) were determined. Aortic root was stained by oil red O (e) and lesion size quantified (f). Aorta was also stained by oil red O (g) and theen facelesion size quantified (h). Hepatic protein levels were determined by western blot assays (i). Scale bar, 200 μm. Values are expressed as mean±s.e.m. Two-sided Student’st-test was performed. *P<0.05, **P<0.01. Figure 5: miR-34a reduces the development of atherosclerosis in Ldlr −/− mice. Ldlr −/− mice were fed a Western diet for a total of 7 weeks ( n =6). At the end of week 4, the mice were injected i.v. with Ad-empty or Ad-miR-34a. Plasma cholesterol ( a ) TG ( b ) cholesterol lipoprotein profile ( c ) and TG lipoprotein profile ( d ) were determined. Aortic root was stained by oil red O ( e ) and lesion size quantified ( f ). Aorta was also stained by oil red O ( g ) and the en face lesion size quantified ( h ). Hepatic protein levels were determined by western blot assays ( i ). Scale bar, 200 μm. Values are expressed as mean±s.e.m. Two-sided Student’s t -test was performed. * P <0.05, ** P <0.01. Full size image p53 and FFAs regulate the miR-34a-HNF4α pathway The finding that the miR-34a-HNF4α pathway is highly induced under common metabolic stress and regulates lipid and lipoprotein metabolism is quite intriguing. However, it remains to be determined which metabolic cue(s) trigger this pathway. p53 is an oxidative stress-inducible protein and is shown to both upregulate miR-34a expression [26] , [27] , [28] , [29] and promote liver steatosis [30] , [31] . Indeed, nuclear p53 protein levels were induced by 6.7-fold in NASH patients ( Fig. 6a,b ). Interestingly, p53 protein levels were unchanged in diabetic mice or HFD-induced mice ( Supplementary Fig. 12a–c ). Overexpression of p53 in HepG2 cells significantly induced miR-34a expression ( Supplementary Fig. 13 ) and reduced HNF4α protein level ( Fig. 6c ). The data of Fig. 6a–c , together with previous observations [26] , [27] , [28] , [29] , [30] , [31] , suggest that p53 may contribute to the induction of the miR-34a-HNF4α pathway and liver steatosis in NASH patients. 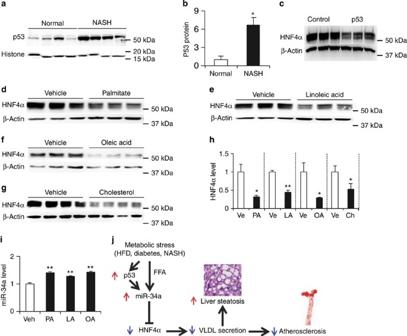Figure 6: p53, fatty acids and cholesterol regulate the miR-34a-HNF4α pathway. (a,b) Nuclear p53 protein levels in the livers of normal individuals and NASH patients were determined by western blot assays (a) and then quantified (b). (c) HepG2 cells were infected with Ad-empty or Ad-p53. After 48 h, protein levels were determined by western blot assays. (d–i) HepG2 cells were treated with either vehicle (Ve), palmitate (PA; 300 μM) (d) linoleic acid (LA; 300 μM) (e) oleic acid (OA; 300 μM) (f) or cholesterol (Ch;10 μg ml−1) (g). Western blot assays were performed (d–g) and then quantified (h). qRT-PCR was used to quantify miR-34a levels (i). (j) Role of the miR-34a-HNF4α pathway in regulating lipid and lipoprotein metabolism. Under metabolic stress, miR-34a is highly induced via both p53-dependent and -independent pathways. The induction of miR-34a causes a reduction in hepatic HNF4α expression and VLDL secretion, leading to liver steatosis and inhibition of atherogenesis. Values are expressed as mean±s.e.m. Two-sided Student’st-test was performed. *P<0.05, **P<0.01. Figure 6: p53, fatty acids and cholesterol regulate the miR-34a-HNF4α pathway. ( a , b ) Nuclear p53 protein levels in the livers of normal individuals and NASH patients were determined by western blot assays ( a ) and then quantified ( b ). ( c ) HepG2 cells were infected with Ad-empty or Ad-p53. After 48 h, protein levels were determined by western blot assays. ( d – i ) HepG2 cells were treated with either vehicle (Ve), palmitate (PA; 300 μM) ( d ) linoleic acid (LA; 300 μM) ( e ) oleic acid (OA; 300 μM) ( f ) or cholesterol (Ch;10 μg ml −1 ) ( g ). Western blot assays were performed ( d–g ) and then quantified ( h ). qRT-PCR was used to quantify miR-34a levels ( i ). ( j ) Role of the miR-34a-HNF4α pathway in regulating lipid and lipoprotein metabolism. Under metabolic stress, miR-34a is highly induced via both p53-dependent and -independent pathways. The induction of miR-34a causes a reduction in hepatic HNF4α expression and VLDL secretion, leading to liver steatosis and inhibition of atherogenesis. Values are expressed as mean±s.e.m. Two-sided Student’s t -test was performed. * P <0.05, ** P <0.01. Full size image Obesity, diabetes and insulin resistance are common risk factors for NAFLD, which is associated with higher levels of free fatty acids (FFAs), cholesterol, insulin and/or glucose in the blood and/or tissues. Treatment of HepG2 cells with palmitate ( Fig. 6d ), linoleic acid ( Fig. 6e ), oleic acid ( Fig. 6f ) or cholesterol ( Fig. 6g ) significantly reduced HNF4α expression ( Fig. 6d–h ). In contrast, insulin or glucose treatment had no effect on HNF4α expression in HepG2 cells ( Supplementary Fig. 14a,b ). Treatment with palmitate, linoleic acid or oleic acid also significantly increased miR-34a expression in HepG2 cells ( Fig. 6i ). Similar results were also observed when the murine primary hepatocytes were used ( Supplementary Fig. 14c–e ). Together, our data suggest that FFAs, cholesterol and p53 are upstream activators for the miR-34a-HNF4α pathway in diabetes, obesity and NASH ( Fig. 6j ). NAFLD is one of the most common liver diseases worldwide. However, the underlying mechanism remains elusive. Here we report that a novel miR-34a-HNF4α pathway regulates both hepatic TG levels and plasma lipid and lipoprotein metabolism. Given that this pathway is activated under common metabolic stress (diabetes, HFD feeding and NASH), this pathway may represent a common mechanism leading to the pathogenesis of human NAFLD. Targeting the miR-34a-HNF4α pathway may be an attractive approach to treatment of NAFLD. The finding that hepatic HNF4α is markedly reduced in diabetes, obesity and NASH is quite intriguing. In NASH patients, hepatic HNF4α protein is almost absent. Consistent with this finding, the vast majority of HNF4α target genes, including those involved in bile acid metabolism, blood coagulation, lipid and lipoprotein metabolism, xenobiotic/drug metabolism and liver differentiation (HNF1α), are significantly reduced in NASH patients ( Supplementary Table 1 ). Previous data show that HNF4α also regulate genes involved in urea synthesis in mice [32] . We do not see any change in genes involved in urea synthesis in NASH patients, which could be due to the difference in species. In HFD-fed mice, hepatic HNF4α protein is reduced only by ∼ 80%. As a result, some of the known Hnf4α target genes are also reduced, whereas some others remain unchanged in these mice ( Supplementary Table 2 ). Other yet-to-be-determined factors may also contribute to the selective regulation of HNF4α target genes in the HFD-fed mice. Previous studies have shown that miR-34a is induced in NAFLD patients [33] , [34] and obese/diabetic mice [35] , [36] . However, whether or how miR-34a regulates hepatic TG metabolism has not been addressed previously. Here we show that increased miR-34a expression results in TG accumulation, whereas inhibition or ablation of miR-34a expression reduces TG accumulation in both mice and HepG2 cells. By using human NASH patient samples and various diabetes and obesity mouse models, we conclude that miR-34a and HNF4α are inversely regulated under all the common metabolic stress. Recently, Lamba et al. [37] also observed a negative correlation between hepatic miR-34a and HNF4α expression in humans, further supporting our finding. The finding that miR-34a inhibits HNF4α expression has led us to hypothesize that miR-34a regulates hepatic TG levels via inhibition of HNF4α. Such a hypothesis is validated by our subsequent studies. Our previous studies demonstrate that loss of hepatic HNF4α has no effect on hepatic TG biosynthesis but causes liver steatosis by reducing VLDL secretion [19] . Consistent with our previous finding, miR-34a reduces VLDL secretion and has no effect on de novo lipogenesis ( Supplementary Fig. 7 ). Thus, our current work not only reveals a novel function for miR-34a in regulating hepatic TG metabolism, but also elucidates how miR-34a regulates hepatic TG metabolism. Choi et al. [38] reported that miR-34a also reduces NAD + levels and SIRT1 activity by targeting NAMPT, the rate-limiting enzyme of NAD + synthesis. Although SIRT1 is known to play an important role in metabolic control, including hepatic TG metabolism, it remains to be determined whether SIRT1 plays a role in miR-34a-regulated TG metabolism. According to our compelling data, miR-34a increases hepatic TG levels by inhibition of HNF4α. Interestingly, overexpression of miR-34a selectively regulates some of the HNF4α target genes ( Fig. 3 ), which could result from incomplete inhibition of HNF4α expression and HNF4α-independent gene regulation. Another important finding of this study is that we demonstrate that the miR-34a-HNF4α pathway also regulates plasma ApoB-containing lipoprotein metabolism and the development of atherosclerosis. Increased plasma levels of ApoB-containing lipoproteins are known to accelerate the development of atherosclerosis. Our data show that the miR-34a-HNF4α pathway promotes hypolipidemia by inhibition of VLDL secretion. In line with this finding, it has been reported that NASH patients have reduced VLDL secretion [39] . As a result of the hypolipidemia, either overexpression of miR-34a or inhibition/ablation of hepatic Hnf4α expression prevents the development of atherosclerosis in Apoe −/− mice or Ldlr −/− mice. These data provide the first evidence demonstrating that the miR-34a-HNF4α pathway regulates the development of atherosclerosis. On the basis of our studies, it will be interesting to investigate whether NASH patients and/or MODY1 patients are protective against atherosclerosis. In addition to elucidating the role of the miR-34a-HNF4α pathway in regulating lipid and lipoprotein metabolism, we also investigated how this pathway is activated under common metabolic stress. Our data suggest that the miR-34a-HNF4α pathway is activated in both p53-dependent and p53-independent manners ( Fig. 6j ). In NASH patients, p53, FFAs and cholesterol may work together to activate the miR-34a-HNF4α pathway. However, p53 is not activated in diabetes or HFD-induced obesity. Thus, under these latter conditions, FFAs and cholesterol may be the major factors triggering activation of the miR-34a-HNF4α pathway. One of our future directions will be to investigate how FFAs and cholesterol activate the miR-34a-HNF4α pathway and whether other metabolic cues are also involved in regulation of this pathway. In summary, the current study has demonstrated that the metabolic stress-inducible miR-34a-HNF4α pathway may play a critical role in both the pathogenesis of NAFLD and regulating plasma lipid and lipoprotein metabolism. Although loss of hepatic HNF4α has a beneficial effect on atherosclerosis and energy homeostasis, loss of hepatic HNF4α causes fatty liver by inhibiting VLDL secretion. Thus, from therapeutic standpoint, suppression of hepatic HNF4α expression together with approaches that alleviate hepatic steatosis may be useful for preventing the development of atherosclerosis. In contrast, overexpression of hepatic HNF4α does not have much effect on plasma lipid or lipoprotein metabolism likely because HNF4α is one of the most abundant genes in the liver [19] . Given that HNF4α expression is markedly reduced under metabolic stress (diabetes, HFD feeding and NASH), delivery of HNF4α via adeno-associated virus or other gene therapy vehicle(s) is a feasible and attractive approach to prevention and treatment of NAFLD associated with metabolic syndrome. In addition, antagonism of hepatic miR-34a function by antagomir(s) is also a feasible approach that may help prevent the development of NAFLD. Thus, targeting the miR-34a-HNF4α pathway represents a promising and attractive approach for treatment of human NAFLD. Human liver tissues, mice and diets C57BL/6, ob / ob , db / db , Hnf4α fl/fl , Ldlr −/− , miR-34a −/− mice and albumin-Cre (Alb-Cre) mice were purchased from the Jackson Laboratories (Bar Harbor, Maine). Hnf4α fl/fl mice were crossed with Ldlr −/− mice to produce Hnf4α fl/fl Ldlr −/− mice, which were subsequently crossed with Alb-Cre mice to produce liver-specific Hnf4α −/− Ldlr −/− ( L - Hnf4α −/− Ldlr −/− ) mice. For streptozotocin (STZ) treatment, C57BL/6J mice were injected intraperitoneally (i.p.) with either vehicle (0.1 M sodium citrate, pH 4.5) or STZ (50 mg kg −1 ) for 5 days and then killed 5 weeks after the treatment. For HFD feeding, C57BL/6J mice were fed a chow diet or an HFD (60% kcal from fat; Research Diets, New Brunswick, NJ, USA) for 16 weeks. For HFHC diet feeding, C57BL/6J mice were fed a chow diet or an HFHC diet (42% kcal fat/0.2% cholesterol; Harlan Teklad, Madison, Wisconsin, USA) for 3 weeks. Unless otherwise stated, male and age-matched (8–12 weeks old) mice were randomly assigned to groups and all mice were fasted for 5-6 h before being killed. Mice that did not look healthy were excluded in the studies. Human liver samples were obtained from the Liver Tissue Cell Distribution System at University of Minnesota. Both male and female individuals were included. The average ages for normal individuals and NASH patients were 55.8 and 52.5 year old, respectively. Individuals with alcohol drinking history (2-3 drinks/day) and liver cancer were excluded from the study. All the animal experiments were approved by the Institutional Animal Care and Use Committee at Northeast Ohio Medical University (NEOMED) and the use of human tissue samples were approved by the Institutional Review Board at NEOMED. Mutagenesis, transfections and cell culture HepG2 cells were purchased from ATCC (Virginia) and cultured in DMEM plus 10% FBS. 3′-UTR of mouse Hnf4α was cloned to the Mlu/PmeI sites of pMIR-Report (catalogue AM5795, Life Technologies). Potential miR-34a binding site A (232-238 nt) and site B (2710-2716 nt) were mutated using a mutagenesis kit from Agilent (catalogue 210518). The forward primer sequences for the mutant binding site A (mutA) and the mutant binding site B (mutB) are 5′-gagaagaccccagggaggactgtcttc ggtctag tggactcctctcaagttgaagtcatcgtc-3′ and 5′-cctaccctgatccccaaggccccaccat ggtctag caagggggtaaaaaagagaaaaagccctc-3′, respectively (mutations are indicated in bold). An miR-34a mimic (C-310529-07-0005) and a control mimic were purchased from Dhmarcon (Thermo Scientific). Transfections were performed using Lipofectamin 2000 (catalogue 11668019, Life Technologies). The miRNA mimics were transfected at a final concentration of 50 nM. For treatment with FAs or cholesterol, HepG2 cells or primary hepatocytes were cultured in serum-free DMEM, then treated with either vehicle or palmitate (300 μM), oleic acid (300 μM), linoleic acid (300 μM) or cholesterol (10 μg ml −1 ). Cells were harvested 48–72 h later for luciferase or western blot assays or lipid extraction. Adenoviruses Ad-shLacZ, Ad-HNF4α, Ad-shHNF4α, Ad-empty (control) and Ad-miR-34a have been described previously [19] , [35] . When Ad-HNF4α was constructed, only the Hnf4α coding region (which does not include any 3′UTR) was cloned into the adenoviral vector. In contrast, Ad-HNF4α-3′UTR, Ad-HNF4α-3′UTR_mutA and Ad-HNF4α-3′UTR_mutB were generated by cloning the Hnf4α coding region plus wild type or mutant 3′UTR (with mutA or mutB) into a pAd/CMV/V5-Dest vector (catalogue V493-20, Life Technologies), followed by transfection into 293 cells for adenovirus production [40] . Ad-p53 was purchased from Vector Biolabs (cat # 1168). Ad-anti-miR-34a was generated by Applied Biological Materials (British Columbia, Canada). Cells were infected with adenoviruses at a multiplicity of infection (MOI) of 5. Mice were intravenously (i.v.) injected with 0.5–1.5 × 10 9 p.f.u. adenoviruses. Unless otherwise stated, the mice were killed 7 days post infection. Real-time PCR RNA was isolated using TRIzol Reagent (Life Technologies, CA). miRNAs were isolated using mirVana miRNA isolation kit (Life Technologies, CA). mRNA levels were determined by quantitative reverse-transcription polymerase chain reaction (qRT-PCR) on a 7500 real-time PCR machine from Applied Biosystems (Foster City, CA) by using SYBR Green Supermix (Roche, Indianapolis, IN). Results were calculated using Ct values and normalized to 36B4 mRNA level. miRNA levels were quantified using TaqMan primers and probes (Catalogue 4427975, Life Technologies, CA) and normalized to U6 levels. MicroRNA Northern blot assays MicroRNA levels were also determined by Northern blot assays following the manufacturer’s instructions (Signosis, Santa Clara, CA. Cat # NB-1001). In the Northern blot assays, robes for miR-34a (Catalogue MP-0602) and U6 (Catalogue MP-0512) were also from Signosis. MTP activity assays Liver was homogenized and MTP activity was measured following the manufacturer’s instructions (Chylos, Inc, Woodbury, NY. Cat #R100). Western blot assays Western blot assays were performed using whole-liver lysates [41] or nuclear proteins of the liver samples and images were collected by ImageQuant LAS 4000 (GE Healthcare, Pittsburgh, PA) [42] . MTP antibody (catalogue sc-135994), HNF4α antibody (catalogue sc-6556) and p53 antibody (catalogue sc-6243) were purchased from Santa Cruz Biotechnology (Santa Cruz, CA). ApoB antibody was purchased from Meridian Life Science (K45253G, TN). β-actin antibody was from Novus Biologicals (catalogue NB600-501, CO). Histone antibody was from Cell Signaling (Beverly, MA). The antibodies were used at a concentration of 1 μg ml −1 . Antagomirs miR-34a LNA inhibitor/antagomir (LNA-miR-34a; anta-miR-34a; anta-34a) and miRNA scramble LNA inhibitor/antagomir (LNA-scr; anta-scr) were synthesized by Exiqon (Denmark, Cat # 199900). ob / ob mice or HFD-fed mice (fed an HF diet for 12 weeks) were injected i.v. with either anta-miR-34a or anta-scr once every 6 days (10 mg kg −1 ). After three injections, mice were killed. Lipid and lipoprotein analysis Approximately 100 mg liver was homogenized in methanol and lipids were extracted in chloroform/methanol (2:1 v/v) as described [43] . Hepatic triglyceride and cholesterol levels were then quantified using Infinity reagents from Thermo Scientific (Waltham, MA). Plasma lipid and glucose levels were also determined using Infinity reagents. Plasma lipoprotein profile was analysed by FPLC as described [19] . In brief, after 100 μl plasma was injected, lipoproteins were run at 0.5 ml min −1 in a buffer containing 0.15 M NaCl, 0.01 M Na 2 HPO4, 0.1 mM EDTA, pH 7.5, and separated on a Superose 6 10/300 GL column (GE Healthcare) by using BioLogic DuoFlow QuadTec 10 System (Bio-Rad, CA). Five hundred microlitres of sample per fraction was collected. VLDL secretion C57BL/6J mice were injected intravenously with specific adenoviruses. On day 6, these mice were fasted overnight, followed by intravenous injection of Tyloxapol (500 mg kg −1 ). Blood was taken at indicated time points and plasma TG levels determined. De novo lipogenesis Mice were injected i.p. with heavy water ( 2 H 2 O) to reach 3% enrichment. After 4 h, livers were collected. Labelled and unlabelled palmitate, glycerol (triglycerides) and cholesterol were analysed by mass spectrometry [19] , [44] . Atherosclerotic lesions The aorta and aortic root were isolated and dissected. The aortic root was washed with phosphate-buffered saline, embedded in optimal cutting temperature compound, and then frozen on dry ice. Serial 7-μm-thick cryosections from the middle portion of the ventricle to the aortic arch were collected on superfrost plus microscope slides (Catalogue 12-550-15, Fisher Scientific). In the region beginning at the aortic valves, every other section was collected. Sectioned aortic root or en face aorta was stained with oil red O and the atherosclerotic lesion size determined using Image-Pro Premier 9.0 (Media Cybernetics, Rockville, MD) [45] . Energy expenditure Mice fed a Western diet were put in the Comprehensive Lab Animal Monitoring System (CLAMS). Oxygen consumption, CO 2 production and heat production were determined [46] . In brief, mice were put in the acclimation cages for 40–48 h. After the acclimation period, mice were weighed and placed back into the acclimation cage with pre-weighed food. Gas exchange was measured in mice every 30 s. Room air was pumped into the mouse calorimetry cages at 0.472–0.600 liters per minute (LPM) and cage air was sampled at 0.4 LPM. Physical activity was measured simultaneously using 16 infrared sensors spread over 19 cm. Data from noon on day 1 to noon on day 2 (EST) were selected for analysis. Statistical analysis Statistical significance was analysed using unpaired two-sided Student’s t -test or ANOVA (GraphPad Prisim, CA). All values are expressed as mean±s.e.m. Differences were considered statistically significant at P <0.05. How to cite this article: Xu Y. et al. A metabolic stress-inducible miR-34a-HNF4α pathway regulates lipid and lipoprotein metabolism. Nat. Commun. 6:7466 doi: 10.1038/ncomms8466 (2015).